UnexpectedE-stereoselective reductive A3-coupling reaction of terminal alkynes with aldehydes and amines The transition-metal catalysed three-component coupling of an alkyne, an aldehyde and an amine has been became a widely used method for preparing propargylic amines. Here, we report an unexpected copper(I)-catalysed E -stereoselective reduction of propargylic amines in situ formed from readily available terminal alkynes, aldehydes and 3-pyrroline or isoindoline via [1,5]-hydride transfer, affording E -allylic amines. Through mechanistic studies, it is believed that the unsaturated cyclic dialkylamine is acting as hydrogen donor. Three-component coupling of an alkyne, an aldehyde and an amine (A 3 -coupling) has been well recognized as a powerful method for the synthesis of propargylic amines ( Fig. 1a ) (refs 1 , 2 , 3 , 4 ). 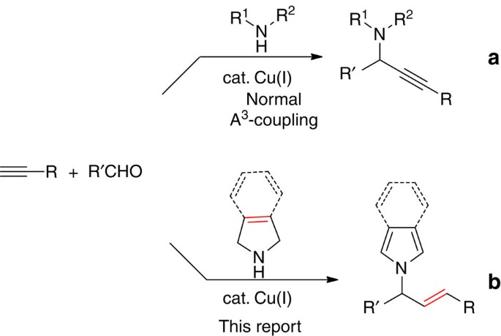Figure 1: Unexpected observation in A3-coupling reactions. (a) A3-coupling for the synthesis of propargylic amines. (b) A3-coupling for the synthesis of allylic amines. During the course of our efforts directed toward the synthesis of functionalized propargylic amines and allenes [5] , [6] , we observed unexpectedly that when treating 2-methybut-3-yn-2-ol 1a with cyclohexanaldehyde 2a and 3-pyrroline in the presence of copper(I) bromide, besides the normal propargylic amine 3aa , the N -allyl pyrrole 4aa was unexpectedly obtained in 42% NMR yield with a complete E -stereoselectivity ( Table 1 , Entry 1). Figure 1: Unexpected observation in A 3 -coupling reactions. ( a ) A 3 -coupling for the synthesis of propargylic amines. ( b ) A 3 -coupling for the synthesis of allylic amines. Full size image Table 1 Optimization of the reaction conditions for 4aa*. Full size table Considering the fact that high E -stereoselective semireduction of a triple bond is an important goal of contemporary organic chemistry [7] , [8] , [9] , [10] , [11] , [12] , [13] , [14] , herein, we wish to report the development of such a highly selective copper(I)-catalysed tandem three-component coupling-semireduction reaction of commercially readily available terminal alkynes, aldehydes and 3-pyrroline or isoindoline affording N -allyl amines with an E -C=C bond ( Fig. 1b ). Optimization of the reaction conditions for 4aa On the basis of these initial observations, we started to work on developing reaction conditions for the exclusive formation of 4aa -type of E -allylic amines ( Table 1 ). When the loading of CuBr was increased to 20 mol%, N -allyl pyrrole 4aa was obtained in 57% NMR yield after 24 h at 25 °C, while the normal A 3 -coupling product propargylic amine 3aa was also formed in 37% yield as determined by NMR analysis ( Table 1 , Entry 2). When the reaction was conducted at 40 °C, 4aa was formed in 84% NMR yield together with 9% NMR yield of the propargylic amine 3aa ( Table 1 , Entry 4). No better result was obtained when further increasing the loading of catalyst at a higher temperature ( Table 1 , Entry 5). Finally, the use of 1.2 equiv of 3-pyrroline provided 4aa as the only product with a higher yield ( Table 1 , Entry 6), which has been defined as the standard reaction conditions for further studies. 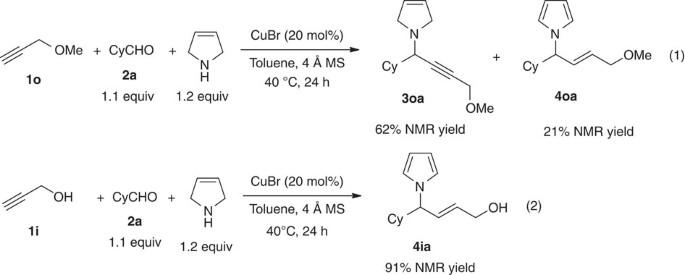Figure 2: Control experiments. (1) The reaction of1owith2aand 3-pyrroline gave a mixture of3oaand4oaunder standard conditions. (2) The reaction of1iwith2aand 3-pyrroline gave4iaas the only product under standard conditions. equiv, equivalent. Substrate scope We next explored the scope of this three-component reaction with representative examples of aldehydes and propargylic alcohols ( Table 2 ). The reaction is quite general: both aliphatic and aromatic aldehydes may all be used with good yields; furthermore, the reaction is not limited to tertiary propargylic alcohols, primary and secondary propargylic alcohols are also good partners for this transformation. In some cases, the reaction requires the addition of CuCl (20 mol%) to ensure complete transformation ( Table 2 , Entries 3, 8 and 12). It is interesting to note that when linear aliphatic aldehydes such as n -hexaldehyde 2c was tested under the standard conditions, the reaction afforded the corresponding product in a low yield with the tentatively assigned 1-(5-((2,5-dihydro-1H-pyrrol-1-yl)methyl)undecan-6-yl)-1H-pyrrole 5c being formed as a byproduct ( Table 2 , Entry 4), which could also be prepared by treating aldehyde 2c with 3-pyrroline in the presence of CuBr in toluene at 40 °C in 82% NMR yield and 7.2/1 dr value. The similar byproduct was also observed using aldehyde 2d . Although side product could not be avoided here, reaction by increasing the loading of aldehyde and 3-pyrroline to 2.0 equivalents can also furnish the desired products in high yield ( Table 2 , Entries 5, 6, 9 and 10). Table 2 Substrate scope*. Full size table Control experiments In order to unveil the role of the hydroxy group, control experiments were conducted. The results in Fig. 2 show a dramatic decrease of reactivity when the hydroxy group was protected as the methyl ether (with 3-methoxyprop-1-yne 1o ). Here, the possible coordination of the hydroxy oxygen may be helping by its coordination with Cu ( Fig. 2 ). Figure 2: Control experiments. (1) The reaction of 1o with 2a and 3-pyrroline gave a mixture of 3oa and 4oa under standard conditions. (2) The reaction of 1i with 2a and 3-pyrroline gave 4ia as the only product under standard conditions. equiv, equivalent. Full size image Synthesis of chiral N -allyl pyrrole ( S )-4aa On the basis of Carreira’s and our previous studies [15] , [16] , [17] , [18] , an efficient synthesis of chiral propargylamine intermediates may be realized. Reaction of propargylic alcohol 1a , aldehyde 2a and 3-pyrroline with CuBr/( R , R )-N-Pinap in toluene afforded the corresponding chiral propargylic amine 4aa in 97% ee. 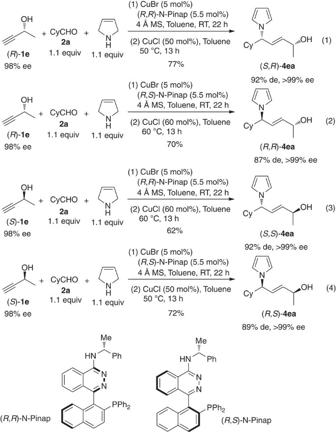Figure 3: Synthesis of four diastereosiomers of 4ea. When a chiral propargylic alcohol was used, we got four diastereosiomers of4eaeasily using either (R,R)-N-Pinap or (R,S)-N-Pinap as the ligand with this protocol. equiv, equivalent. Interestingly, it should be noted that the second-step reaction with CuBr was very slow ( Table 3 , Entries 1 and 2). Subsequent transformation of the crude propargylic amine 4aa was conducted in the same solvent in the presence of CuCl affording the chiral N -allyl pyrrole 4aa with 63% yield and 97% ee ( Table 3 , Entry 6). Table 3 Initial efforts to synthesize chiral N -allyl pyrrole (S)-4aa*. Full size table Synthesis of four diastereosiomers of 4ea When the optically active propargylic alcohols with a central chirality such as ( R )- 1e and ( S )- 1e were used, all four isomers ( S , R )-4ea , ( R , R )-4ea , ( S , S )-4ea and ( R , S )-4ea were obtained successfully with this protocol using either ( R , R )- N -Pinap or ( R , S )- N -Pinap as the ligand (Equations 1–4, Fig. 3 ). The absolute configurations of N -allyl pyrrole were assigned based on our previous report [5] . Figure 3: Synthesis of four diastereosiomers of 4ea. When a chiral propargylic alcohol was used, we got four diastereosiomers of 4ea easily using either ( R , R )- N -Pinap or ( R , S )- N -Pinap as the ligand with this protocol. equiv, equivalent. Full size image Reaction with normal terminal alkynes However, the reaction could not be extended to normal terminal alkynes under this set of standard reaction conditions. 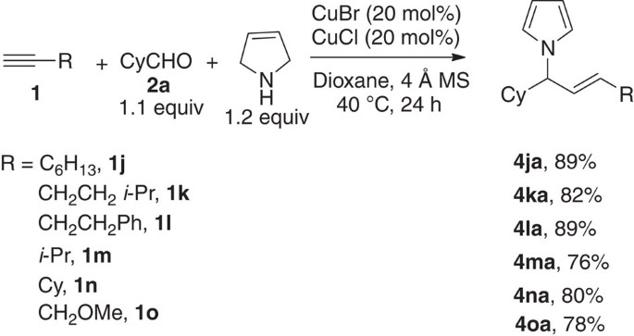Figure 4: Reaction with simple non-functionalized terminal alkynes. The reaction of various simple terminal alkynes with2aand 3-pyrroline gaveN-allyl pyrrole4in good yields with the combination of CuBr and CuCl in dioxane. equiv, equivalent. After numerous trials and errors ( Table 4 ), luckily, we observed that the reaction with alkyne 1j , cyclohexanaldehyde 2a and 3-pyrroline proceeds very efficiently in 1,4-dioxane with the combination of CuBr and CuCl affording N -allyl pyrrole 4ja in 89% yield. Some extra examples are shown in Fig. 4 . Here, the reaction of 3-methoxyprop-1-yne 1o could also perform well under this set of conditions. Table 4 Optimization of the reaction conditions with normal terminal akynes*. Full size table Figure 4: Reaction with simple non-functionalized terminal alkynes. The reaction of various simple terminal alkynes with 2a and 3-pyrroline gave N -allyl pyrrole 4 in good yields with the combination of CuBr and CuCl in dioxane. equiv, equivalent. Full size image Reaction with isoindoline Furthermore, isoindoline may also be used with N- allyl isoindole 6 being formed in 91% NMR yield, which was characterized by converting to 7 in 70% combined yield by a Diels–Alder reaction with N -methylmaliemide ( Fig. 5 ). 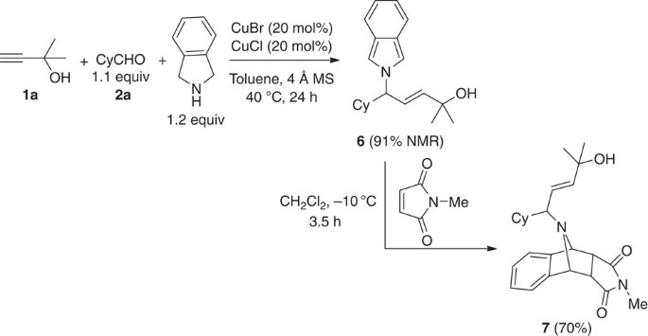Figure 5: A reaction with isoindoline. The reaction of isoindoline with1aand2aaffordedN-allyl isoindole6, which was converted to7by Diels–Alder reaction withN-methylmaliemide. equiv, equivalent. Figure 5: A reaction with isoindoline. The reaction of isoindoline with 1a and 2a afforded N- allyl isoindole 6 , which was converted to 7 by Diels–Alder reaction with N -methylmaliemide. equiv, equivalent. Full size image To provide further insight into the reaction mechanism, deuterium-labeling experiments were performed as depicted in Fig. 6 . Deuterium-labeled d 4 -3b (96% d -incorporation), prepared from o -phthalimide (Equation 1, Fig. 6 ), was treated with CuCl in toluene at 60 °C for 24 h giving d 4 - 6 in 61% NMR yield. 1 H NMR studies of the crude product d 4 - 6 show that the d -incorporation at γ-position of N- allyl isoindole 6 was 92%, indicating an intramolecular 1,5-hydride transfer from the deuterated isoindole unit. The low D-incorporation at the β-position (17%) was obviously caused by the presence of the free OH group in the terminal propargylic alcohol 1a (Equation 2, Fig. 6 ). The reaction of deuterium-labeled d 4 -3c (96% d -incorporation) in the presence of CuBr and CuCl in dioxane at 90 °C gave d 4 - 8 in poor NMR yield (32%) with only 17% D-incorporation at the β-position, suggesting the external proton source participated in the protodemetalation (Equation 3, Fig. 6 ). Compounds 3c and d 4 -3c were then treated under similar conditions in the presence of 10.0 equivalents of CH 3 COOD, affording a 78% NMR yield of d 1 - 8 with 52% D-incorporation at the β-position and a 60% NMR yield of d 4 - 8 with 81% D-incorporation at the β-position (93% D-incorporation at the γ-position), respectively (Equations 4 and 5, Fig. 6 ), reconfirming that the β-position proton may be from the azacycle and the moisture in ambient environment. The low D-incorporation in the isoindole unit in d 4 - 8 was caused by the facile H/D exchange as confirmed by the results shown in Equation 6. 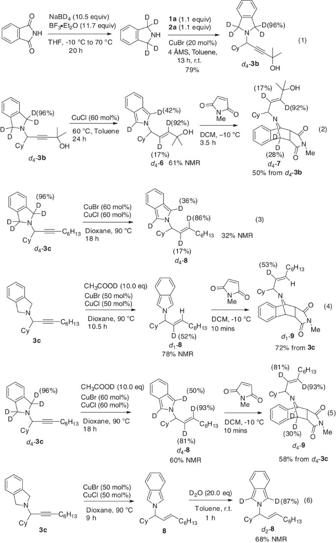Figure 6: Deuterium-labeling experiments. (1) Preparation of deuterium-labeled propargylic amined4-3b. (2) Reaction ofd4-3bgaved4-6. (3) Reaction ofd4-3cgivingd4-8. (d) Reaction of3cemploying AcOD givingd1-8. (e) Reaction ofd4-3cemploying AcOD givingd4-8. (f) Reaction of8with D2O givingd2-8. equiv, equivalent. Figure 6: Deuterium-labeling experiments. (1) Preparation of deuterium-labeled propargylic amine d 4 -3b . (2) Reaction of d 4 -3b gave d 4 - 6 . (3) Reaction of d 4 -3c giving d 4 - 8 . (d) Reaction of 3c employing AcOD giving d 1 - 8 . (e) Reaction of d 4 -3c employing AcOD giving d 4 - 8 . (f) Reaction of 8 with D 2 O giving d 2 - 8 . equiv, equivalent. Full size image On the basis of these results, we propose a mechanism for this unique unexpected A 3 -coupling-stereodefined reduction reaction as shown in Fig. 7 . The reaction of CuBr with the propargylic alcohol generates the copper alkynylide species 10 , which would then react with the iminium intermediate 11 formed in situ from the aldehyde and isoindoline to yield the corresponding propargylic amine-CuBr complex 12 . This compound would afford, via an anti-1,5-hydride transfer process, the iminium intermediate 13 , which would undergo protodemtalation with H + or D + readily to afford the N -allyl isoindole product d 4 - 6 and regenerate the copper catalyst due to the aromatization of the azacycle ( Fig. 7 ). 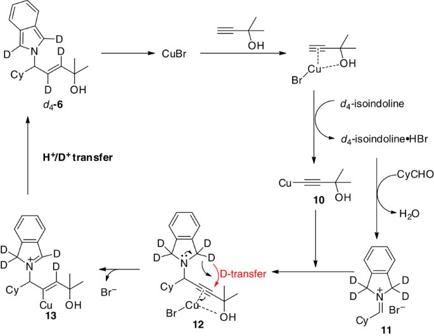Figure 7: Proposed mechanism for CuBr-catalysed A3-coupling/reduction reaction. The key step is the formation of propargylic amines followed by 1,5-Hydride transfer, aromatization and protodemtalation. Figure 7: Proposed mechanism for CuBr-catalysed A 3 -coupling/reduction reaction. The key step is the formation of propargylic amines followed by 1,5-Hydride transfer, aromatization and protodemtalation. Full size image In conclusion, we have developed a copper(I)-catalysed three-component tandem reaction for the synthesis of N -allyl pyrroles. This novel reaction is simple and atom economic, affording N -allyl pyrroles with exclusive E -stereoselectivity under exceptionally mild conditions. Moreover, it could provide a highly attractive and convergent approach toward optically active N -allyl amines efficiently. Further investigation including the synthetic application is currently ongoing in our laboratory. Materials All reactions have been carried out in oven-dried Schlenk tubes. CuBr (98%) and CuCl were purchased from Acros and kept in glove box; ( R,R )- N -Pinap (97%) and ( R,S )- N -Pinap (97%) were purchased from Stream Chemicals and kept in glove box; 4 Å molecular sieves was purchased from Alfa Aesar and kept in glove box after activation (heated at 450 °C for 10 h in Muffle furnace, taken out after cooling to 200 °C and then kept in a glove box to allow to cool to room temperature). 3-Pyrroline (96%) was purchased from Alfa. Isoindoline (98%) was purchased from TCI. Aldehydes were distilled right before use. Toluene, 1,4-dioxane and tetrahydrofuran were dried over sodium wire with benzophenone as the indicator and distilled freshly before use. Other reagents were used as received without further treatment. All the temperatures are referred to the oil baths used. General spectroscopic methods 1 H NMR spectra were obtained at 20 °C using a Bruker spectrometer operating at 300 MHz. 13 C NMR spectra were obtained at 20 °C using a Bruker spectrometer operating at 75 MHz. 1 H NMR, 13 C NMR and high-performance liquid chromatography spectra are supplied for all compounds: see Supplementary Figs 1–90 . See Supplementary Methods for the characterization data of compounds not listed in this part. Synthesis of compound 4aa To a flame-dried Schlenk tube were added CuBr (98% purity, 29.5 mg, 0.2 mmol) and 4 Å molecular sieves (300.7 mg) inside a glove box. 1a (84.5 mg, 1.0 mmol)/toluene (1.0 ml), 2a (122.9 mg, 1.1 mmol)/toluene (1.0 ml) and 3-pyrroline (96% purity, 86.7 mg, 1.2 mmol)/toluene (1.0 ml) were then added sequentially under Ar atmosphere. The Schlenk tube was then stirred at 40 °C until completion of the reaction as monitored by thin-layer chromatography (TLC; 24 h). The crude reaction mixture was filtered through a short pad of silica gel eluted with ether (30 ml). After evaporation, the residue was purified by chromatography on silica gel to afford 4aa (219.4 mg, 88%; eluent: petroleum ether/ethyl acetate=20/1 to 10/1) as a liquid: 1 H NMR (300 MHz, CDCl 3 ) δ =6.66 (t, J =2.0 Hz, 2 H, from pyrrolyl), 6.14 (t, J =2.1 Hz, 2 H, from pyrrolyl), 5.85 (dd, J 1 =15.6 Hz, J 2 =8.1 Hz, 1 H, one proton from CH=CH), 5.68 (d, J =15.6 Hz, 1 H, one proton from CH=CH), 4.00 (t, J =8.6 Hz, 1 H, NCHC=C), 1.83–1.58 (m, 5 H, protons from Cy), 1.49 (s, 1 H, OH), 1.35–1.05 (m, 10 H, protons from Cy and OC(CH 3 ) 2 ), 0.99–0.75 (m, 2 H, protons from Cy); 13 C NMR (75 MHz, CDCl 3 ) δ =141.0, 125.3, 119.2, 107.4, 70.6, 67.3, 43.0, 30.3, 29.8, 29.6, 26.2, 25.93, 25.87; mass spectrometry (electrospray ionization) (MS (ESI)) m/z=248 (M+H + ); infrared (IR; neat): v =3,331, 2,972, 2,930, 2,849, 1,488, 1,447, 1,403, 1,377, 1,359, 1,336, 1,320, 1,264, 1,225, 1,185, 1,143, 1,091, 1,064, 1,054 cm −1 ; high-resolution mass spectrometry (HRMS) calculated for C 16 H 26 NO [M+H + ]: 248.2009, found: 248.2006. Synthesis of compound ( S )- 4aa To a flame-dried Schlenk tube were added CuBr (98% purity, 3.6 mg, 0.025 mmol) and ( R,R )- N -Pinap (97% purity, 15.8 mg, 0.0275, mmol) inside a glove box. The Schlenk tube was taken out, toluene (1 ml) was then added under Ar atmosphere. The Schlenk tube was then stirred at room temperature for 1 h. 4 Å molecular sieves (150.1 mg), 1a (42.0 mg, 0.5 mmol)/toluene (0.5 ml), 2a (61.8 mg, 0.55 mmol)/toluene (0.5 ml) and 3-pyrroline (96% purity, 39.7 mg, 0.55 mmol)/toluene (0.5 ml) were then added sequentially under Ar atmosphere. The Schlenk tube was then stirred at room temperature until completion of the reaction as monitored by TLC (22 h). The crude reaction mixture was filtered through a short pad of silica gel eluted with ether (30 ml). After evaporation, the residue was filtered through a short column of silica gel (eluent: petroleum ether/ethyl acetate/Et 3 N=250/50/0.13 ml) to collect the crude propargylic amine ( S )- 3aa after evaporation, which was used in the next step directly. To another Schlenk tube was added CuCl (24.8 mg, 0.25 mmol) inside a glove box; the above crude product was then dissolved in toluene (5.0 ml) and transferred to the Schlenk tube under Ar atmosphere. The Schlenk tube was then stirred at 50 °C until completion of the reaction as monitored by TLC (14 h). The crude reaction mixture was filtrated through a short pad of silica gel eluted with ether (30 ml). After evaporation, the residue was purified by chromatography on silica gel to afford ( S )- 4aa (77.4 mg, 63%; 5% of ( S )- 3aa was observed by NMR analysis of crude product; eluent: petroleum ether/ethyl acetate=20/1 to 10/1) as a liquid: 97% ee (high-performance liquid chromatography conditions: Chiralcel AD-H column, hexane/ i -PrOH=200/1, 1.0 ml min −1 , λ =214 nm, t R (major)=41.5 min, t R (minor) =46.1 min); [α] D 24 =+62.8 ( c =1.08, CHCl 3 ); 1 H NMR (300 MHz, CDCl 3 ) δ =6.65 (t, J =2.2 Hz, 2 H, from pyrrolyl), 6.13 (t, J =2.1 Hz, 2 H, from pyrrolyl), 5.84 (dd, J 1 =15.6 Hz, J 2 =8.1 Hz, 1 H, one proton from CH=CH), 5.68 (d, J =15.6 Hz, 1 H, one proton from CH=CH), 4.00 (t, J =8.6 Hz, 1 H, NCHC=C), 1.82–1.58 (m, 6 H, protons from Cy and OH), 1.35–1.05 (m, 10 H, protons from Cy and OC(CH 3 ) 2 ), 0.97–0.74 (m, 2 H, protons from Cy); 13 C NMR (75 MHz, CDCl 3 ) δ =141.0, 125.3, 119.2, 107.4, 70.6, 67.3, 43.0, 30.3, 29.8, 29.6, 26.2, 25.94, 25.88; MS (ESI) m/z=248 (M+H + ); IR (neat): v =3,379, 2,971, 2,923, 2,852, 1,487, 1,449, 1,405, 1,362, 1,318, 1,263, 1,230, 1,186, 1,150, 1,088, 1,065 cm −1 ; HRMS calculated for C 16 H 26 NO [M+H + ]: 248.2009, found: 248.2010. Synthesis of compound 4ja To a flame-dried Schlenk tube were added CuBr (98% purity, 29.8 mg, 0.2 mmol), CuCl (19.8 mg, 0.2 mmol) and 4 Å molecular sieves (300.1 mg) inside a glove box. 1j (98% purity, 112.6 mg, 1.0 mmol)/dioxane (1.0 ml), 2a (124.0 mg, 1.1 mmol)/dioxane (1.0 ml) and 3-pyrroline (96% purity, 87.0 mg, 1.2 mmol)/dioxane (1.0 ml) were then added sequentially under Ar atmosphere. The Schlenk tube was then stirred at 40 °C until completion of the reaction as monitored by TLC analysis (24 h). The crude reaction mixture was filtered through a short pad of silica gel eluted with ether (30 ml). After evaporation, the residue was purified by chromatography on silica gel to afford 4ja (244.3 mg, 89%; eluent: petroleum ether/ethyl acetate=100/1) as a liquid: 1 H NMR (300 MHz, CDCl 3 ) δ =6.65 (t, J =2.2 Hz, 2 H, from pyrrolyl), 6.12 (t, J =2.1 Hz, 2 H, from pyrrolyl), 5.67–5.47 (m, 2 H, CH=CH), 3.97 (t, J =8.2 Hz, 1 H, NCHC=C), 2.06–1.95 (m, 2 H, C=CCH 2 ), 1.83–1.58 (m, 5 H, protons from Cy), 1.41–1.05 (m, 12 H, protons from Cy and four CH 2 ), 0.96–0.74 (m, 5 H, protons from Cy and CH 3 ); 13 C NMR (75 MHz, CDCl 3 ) δ =134.1, 128.4, 119.0, 107.2, 67.8, 43.0, 32.3, 31.6, 30.2, 29.7, 29.0, 28.8, 26.3, 26.0, 25.9, 22.6, 14.0; MS (ESI) m/z=274 (M+H + ); IR (neat): v =2,924, 2,853, 1,487, 1,449, 1,264, 1,089 cm −1 ; HRMS calculated for C 19 H 32 N [M+H + ]: 274.2529, found: 274.2527. Synthesis of compound 7 To a flame-dried Schlenk tube were added CuBr (98% purity, 29.8 mg, 0.2 mmol), CuCl (19.6 mg, 0.2 mmol) and 4 Å molecular sieves (300.0 mg) inside a glove box. 1a (83.8 mg, 1.0 mmol)/toluene (1.0 ml), 2a (123.7 mg, 1.1 mmol)/toluene (1.0 ml) and isoindoline (98% purity, 146.4 mg, 1.2 mmol)/toluene (1.0 ml) were then added sequentially under Ar atmosphere. The Schlenk tube was then stirred at 40 °C until completion of the reaction as monitored by TLC (24 h). The crude reaction mixture was filtered through a short pad of silica gel eluted with ether (30 ml). After evaporation, the crude product 6 was used in the next step without further treatment. The crude product 6 was dissolved in 5 ml of CH 2 Cl 2 in a Schlenk tube. A solution of N -methylmaleimide (122.4 mg, 1.1 mmol) in 5 ml of CH 2 Cl 2 was added via a syringe over 5 min at −10 °C. The Schlenk tube was then stirred at this temperature until completion of the reaction as monitored by TLC (3.5 h). After evaporation, the residue was purified by chromatography on silica gel to afford 7 (285.7 mg, 70%; eluent: petroleum ether/ethyl acetate=2/1) as a liquid: 1 H NMR (300 MHz, CDCl 3 ) δ =7.27–7.13 (m, 4 H, Ar–H), 5.51–5.44 (m, 2 H, CH=CH), 4.76 (d, J =4.5 Hz, 1 H, NCHAr), 4.69 (d, J =4.8 Hz, 1 H, NCHAr), 3.68–3.57 (m, 2 H, 2 × CHC=O), 2.35 (q, J =3.9 Hz, 1 H, NCH–C=C), 2.25 (s, 3 H, O=C–NCH 3 ), 1.90–1.60 (m, 5 H, protons from Cy and OH), 1.48–0.75 (m, 13 H, protons from Cy and OC(CH 3 ) 2 ); 13 C NMR (75 MHz, CDCl 3 ) δ =176.1, 176.0, 141.7, 140.4, 139.8, 127.5, 127.4, 124.4, 122.8, 122.6, 70.5, 65.5, 64.7, 63.4, 47.3, 46.8, 40.4, 30.9, 29.9, 29.7, 26.6, 26.5, 26.4, 23.63, 23.61; MS (ESI) m/z=409 (M+H + ); IR (neat): v =3,453, 2,924, 2,852, 1,774, 1,693, 1,433, 1,378, 1,286, 1,235, 1,206, 1,126, 1,064 cm −1 ; HRMS calculated for C 25 H 33 N 2 O 3 [M+H + ]: 409.2486, found: 409.2489. Synthesis of compound d 4 - 3b To a flame-dried 250 ml three-necked flask was added o -phthalimide (1.2941, g, 8.8 mmol), tetrahydrofuran (90 ml) and sodium tetradeuteridoborate (3.8513, g, 92.0 mmol) sequentially under Ar atmosphere. After being cooled to −10 °C, BF 3 ·Et 2 O (12.7 ml, d=1.15 g ml −1 , 102.6 mmol) was added slowly via a syringe. Once the addition was complete, the reaction mixture was heated at 70 °C with stirring. After 20 h, the reaction mixture was allowed to cool to 0 °C, quenched slowly with cold water (18 ml), diluted with ethyl acetate (140 ml) and adjusted pH value to 10 using an aqueous solution of NaOH (6.0 M). The organic layer was separated, washed with brine (4 × 70 ml) and dried over anhydrous Na 2 SO 4 . Solvent was removed in vacuo . The residual green solid was diluted with diethyl ether (50 ml) and acidified to pH 2 using an aqueous solution of HCl (6.0 M) with stirring at 0 °C. The aqueous layer was separated, adjusted pH value to 10 using an aqueous solution of NaOH (6.0 M) at 0 °C and extracted with ethyl acetate (100 ml). The organic layer was separated, washed with brine (3 × 70 ml), dried over anhydrous Na 2 SO 4 and rotary evaporated to give the crude d 4 -isoindoline (431.2 mg) as an oil, which was used in the next step without further treatment. To a flame-dried Schlenk tube were added CuBr (98% purity, 103.1 mg, 0.7 mmol) and 4 Å molecular sieves (1.0002, g) inside a glove box. 1a (328.9 mg, 3.9 mmol)/toluene (2.0 ml), 2a (437.7 mg, 3.9 mmol)/toluene (2.0 ml) and the crude d 4 -isoindoline (431.2 mg, 3.5 mmol)/toluene (6.0 ml) were then added sequentially under Ar atmosphere. The Schlenk tube was then stirred at room temperature until completion of the reaction as monitored by TLC (13 h). The crude reaction mixture was filtered through a short pad of silica gel eluted with ether (50 ml). After evaporation, the residue was purified by chromatography on silica gel to afford d 4 -3b (831.3 mg, 79%) as a liquid: 1 H NMR (300 MHz, CDCl 3 ) δ =7.21–7.12 (m, 4 H, Ar–H), 3.31 (d, J =9.0 Hz, 1 H, CHC≡C), 2.41 (bs, 1 H, OH), 2.10–1.94 (m, 2 H, protons from Cy), 1.81–1.62 (m, 3 H, protons from Cy), 1.57–1.39 (m, 7 H, protons from Cy and OC(CH 3 ) 2 ), 1.35–0.94 (m, 5 H, protons from Cy); 1 H NMR (300 MHz, CDCl 3 ), the following signal is discernible for 3b : δ =3.97 (d, J =11.4 Hz, 0.17 H, two NCH 2 ); 13 C NMR (75 MHz, CDCl 3 ) δ =139.7, 126.4, 122.2, 92.4, 79.2, 65.0, 60.1, 54.4 (quint, J C–D =20.7 Hz), 40.9, 31.7, 31.6, 30.3, 30.2, 26.5, 26.02, 25.97; MS (ESI) m/z=302 (M+H + ); IR (neat): v =3,395, 2,979, 2,923, 2,851, 2,788, 1,464, 1,449, 1,362, 1,223, 1,165, 1,133, 1,069 cm −1 ; HRMS calculated for C 20 H 24 D 4 NO [M+H + ]: 302.2416, found: 302.2418. Synthesis of compound d 4 - 7 To a flame-dried Schlenk tube were added CuCl (77.0 mg, 0.77 mmol) inside a glove box. d 4 -3b (386.8 mg, 1.28 mmol)/toluene (5 ml) were then added sequentially under Ar atmosphere. The Schlenk tube was then stirred at 60 °C until completion of the reaction as monitored by TLC (24 h). The crude reaction mixture was filtered through a short pad of silica gel eluted with ether (30 ml). After evaporation, the crude product d 4 -6 was used in the next step without further treatment. 1 H NMR analysis of the crude d 4 -6 showed occurrence of 92% and 17% deuteration at γ-position and β-position of N -allylisoindole 6 . The crude product d 4 -6 was dissolved in 6 ml of CH 2 Cl 2 in a Schlenk tube. A solution of N -methylmaleimide (97.8 mg, 0.88 mmol) in 4 ml of CH 2 Cl 2 was added via a syringe over 5 min at −10 °C. The Schlenk tube was then stirred at this temperature until completion of the reaction as monitored by TLC (3.5 h). After evaporation, the residue was purified by chromatography on silica gel to afford d 4 -7 (262.5 mg, 50%; eluent: petroleum ether/ethyl acetate=2/1) as a liquid: 1 H NMR (400 MHz, CDCl 3 ) δ =7.27–7.13 (m, 4 H, Ar–H), 3.68–3.58 (m, 2 H, two CHC=O), 2.40–2.30 (m, 1 H, NCH–C=C), 2.25 (s, 3 H, NCH 3 ), 2.05–1.60 (m, 5 H, protons from Cy and OH), 1.48–0.79 (m, 13 H, protons from Cy and OC(CH 3 ) 2 ); 1 H NMR (400 MHz, CDCl 3 ), the following signal is discernible for 7 : δ =5.51–5.44 (m, 0.9 H, CH=CH), 4.76 (d, J =4.4 Hz, 0.72 H, NCHAr), 4.70 (d, J =4.0 Hz, 0.72 H, NCHAr); MS (ESI) m/z=413 (M+H + ). Synthesis of compound d 4 - 9 To a flame-dried Schlenk tube were added CuCl (29.5 mg, 0.3 mmol) and CuBr (98% purity, 43.7 mg, 0.3 mmol) inside a glove box. d 4 -3c (163.0 mg, 0.5 mmol)/dioxane (3 ml) and CH 3 COOD (288 μl, d =1.059 g ml −1 , 5.0 mmol) were then added sequentially under Ar atmosphere. The Schlenk tube was then stirred at 90 °C until completion of the reaction as monitored by TLC (18 h). The crude reaction mixture was filtered through a short pad of silica gel eluted with toluene (30 ml). After evaporation, the crude product d 4 - 8 was used in the next step without further treatment. 1 H NMR analysis of the crude d 4 -8 showed occurrence of 93% and 81% deuteration at γ-position and β-position of N -allylisoindole 8 . The crude product d 4 - 8 was dissolved in 2.5 ml of CH 2 Cl 2 in a Schlenk tube. A solution of N -methylmaleimide (37.0 mg, 0.33 mmol) in 2.5 ml of CH 2 Cl 2 was added via a syringe over 5 min at −10 °C. The Schlenk tube was then stirred at this temperature until completion of the reaction as monitored by TLC (10 min). After evaporation, the residue was purified by chromatography on silica gel to afford d 4 - 9 (126.0 mg, 58%; eluent: petroleum ether/ethyl acetate=10/1) as a liquid: 1 H NMR (300 MHz, CDCl 3 ) δ =7.26–7.11 (m, 4 H, Ar–H), 3.67–3.57 (m, 2 H, 2 × CHC=O), 2.35-2.27 (m, 1 H, NCH–C=C), 2.24 (s, 3 H, NCH 3 ), 2.08–1.95 (m, 2 H, C=CCH 2 ), 1.90–1.60 (m, 4 H, protons from Cy), 1.46–0.82 (m, 18 H, protons from Cy, 4 × CH 2 and CH 3 ); 1 H NMR (300 MHz, CDCl 3 ), the following signal is discernible for 9 : δ =5.36–5.20 (m, 0.26 H, CH=CH), 4.79–4.69 (m, 1.39 H, 2 × NCHAr). How to cite this article: Fan, W. et al. Unexpected E -stereoselective reductive A 3 -coupling reaction of terminal alkynes with aldehydes and amines. Nat. Commun. 5:3884 doi: 10.1038/ncomms4884 (2014).